Decreased extra-renal urate excretion is a common cause of hyperuricemia ABCG2, also known as BCRP, is a high-capacity urate exporter, the dysfunction of which raises gout/hyperuricemia risk. Generally, hyperuricemia has been classified into urate 'overproduction type' and/or 'underexcretion type' based solely on renal urate excretion, without considering an extra-renal pathway. Here we show that decreased extra-renal urate excretion caused by ABCG2 dysfunction is a common mechanism of hyperuricemia. Clinical parameters, including urinary urate excretion, are examined in 644 male outpatients with hyperuricemia. Paradoxically, ABCG2 export dysfunction significantly increases urinary urate excretion and risk ratio of urate overproduction. Abcg2 -knockout mice show increased serum uric acid levels and renal urate excretion, and decreased intestinal urate excretion. Together with high ABCG2 expression in extra-renal tissues, our data suggest that the 'overproduction type' in the current concept of hyperuricemia be renamed 'renal overload type', which consists of two subtypes—'extra-renal urate underexcretion' and genuine 'urate overproduction'—providing a new concept valuable for the treatment of hyperuricemia and gout. Hyperuricemia induces gout and kidney stones and accelerates the progression of renal and cardiovascular diseases [1] , [2] . Unlike other mammals, hominoids, including humans, show high serum uric acid levels (SUAs), because uric acid (urate) is the end product in the purine metabolism owing to the lack of the urate-degrading enzyme uricase [3] . It is commonly accepted that two-thirds of the urate is excreted from the kidney into urine via the 'renal excretion' pathway, and the remaining third via the 'extra-renal excretion' pathway, such as gut excretion [4] , [5] . Hyperuricemia has been clinically classified into the urate 'overproduction' type, the 'underexcretion' type, and the 'combined' type. This classification is, however, based solely on the amount of renal urate excretion and urate clearance [6] , [7] , [8] , [9] , and extra-renal excretion, for example, via the gut excretion pathway, is not considered. The kidney has been recognized as a main regulator of SUA and renal urate excretion is determined by the balance of the reabsorption and secretion of urate. Renal urate reabsorption is mainly mediated by two urate transporters; urate transporter 1 (URAT1, also known as SLC22A12) [10] and glucose transporter 9 (GLUT9, also known as SLC2A9 (refs 11 , 12 , 13 , 14 , 15 )). Recent genome-wide association studies of SUA identified the involvement of several transporter genes including ATP-binding cassette transporter, sub-family G, member 2 ( ABCG2 , also known as BCRP [16] , [17] , [18] ). The ABCG2 gene locates in a gout-susceptibility locus on chromosome 4q, which was previously demonstrated by a genome-wide linkage study of gout [19] . Woodward et al . and our group independently found that ABCG2 transports urate and shows the reduced urate transport by a half-functional variant, Q141K (rs2231142) [20] , [21] . In addition, ABCG2 has been identified as a high-capacity urate exporter that would mediate renal and/or extra-renal urate excretion [21] . We also showed that common dysfunctional genotype combinations of ABCG2 gene (Q126X (rs72552713) and Q141K) are a major cause of gout [21] . In this study, we investigated the relationship between ABCG2 dysfunction and urate excretion in hyperuricemia patients and mouse model. We found that decreased extra-renal urate excretion is a common cause of hyperuricemia, which has not been considered in the current pathophysiological concept of hyperuricemia. Renal urate excretion in hyperuricemia patients We investigated the relationship between ABCG2 dysfunction and renal urate excretion in hyperuricemia patients in this study. The characteristics and genotypes of the participants are summarized in Supplementary Tables S1 and S2 , respectively. The patients' types of hyperuricemia were determined according to the classification of hyperuricemia ( Fig. 1 ), which is based on the patient's urinary urate excretion (UUE) and fractional excretion of urate clearance (urate clearance/creatinine clearance ratio, FE UA ). The risk allele frequency of Q126X (risk allele, X) and Q141K (risk allele, K), among 644 male outpatients with hyperuricemia including 575 gout cases, was 4.1 and 45.9%, respectively. Those who had Q126X and Q141K variants were 8.1 and 71.9%, respectively, of all patients ( Supplementary Table S2 ). Subsequent haplotype frequency analysis revealed that the minor alleles of Q126X and Q141K were in different haplotypes ( Supplementary Table S3 ), which indicated that these variants were independent risks, as reported previously [21] . Therefore, we could estimate urate export function of ABCG2 by the combination of two common variants, non-functional Q126X and half-functional Q141K ( Supplementary Fig. S1 ). Patients were then divided into four groups by genetically estimated ABCG2 function [21] ; that is, full function, 3/4 function (mild dysfunction), 1/2 function (moderate dysfunction) and ≤1/4 function (severe dysfunction) ( Supplementary Table S4 ). Altogether, 75.6% of all patients had ABCG2 dysfunction. 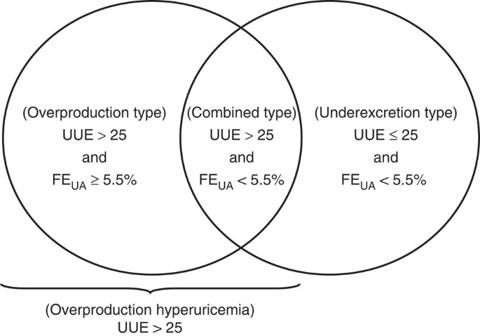Figure 1: Current classification of hyperuricemia. Classification of hyperuricemia is based on UUE and fractional excretion of urate (FEUA). In this study, patients were classified as overproduction hyperuricemia, when their UUE was over 25.0 mg h−1/1.73 m2(600 mg per day/1.73 m2). Those who had FEUAunder 5.5% were classified as underexcretion hyperuricemia. Combined type was classified when their UUE and FEUAmet the criteria of both overproduction and underexcretion hyperuricemia. Patients who met the single criterion of overproduction hyperuricemia, excluding combined type, were defined as overproduction type. In addition to the types shown in this figure, there is a 'normal type' whose UUE is ≤25 mg h−1/1.73 m2and FEUAis ≥5.5%. UUE unit, mg h−1/1.73 m2. Figure 1: Current classification of hyperuricemia. Classification of hyperuricemia is based on UUE and fractional excretion of urate (FE UA ). In this study, patients were classified as overproduction hyperuricemia, when their UUE was over 25.0 mg h −1 /1.73 m 2 (600 mg per day/1.73 m 2 ). Those who had FE UA under 5.5% were classified as underexcretion hyperuricemia. Combined type was classified when their UUE and FE UA met the criteria of both overproduction and underexcretion hyperuricemia. Patients who met the single criterion of overproduction hyperuricemia, excluding combined type, were defined as overproduction type. In addition to the types shown in this figure, there is a 'normal type' whose UUE is ≤25 mg h −1 /1.73 m 2 and FE UA is ≥5.5%. UUE unit, mg h −1 /1.73 m 2 . 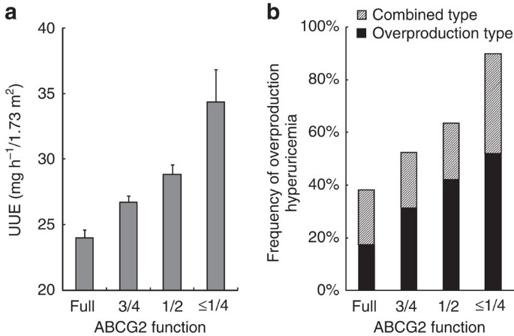Figure 2: Increase of UUE and the frequency of overproduction hyperuricemia by ABCG2 dysfunction. (a) UUE according to each ABCG2 function (n=644). Patients with hyperuricemia were divided into four groups by their estimated ABCG2 functions, that is, full function, 3/4 function, 1/2 function and ≤1/4 function. UUE showed an inverse association with ABCG2 functions (P=3.60×10−10by simple linear regression analysis). All bars show mean±s.e.m. (b) Frequency of 'overproduction' hyperuricemia according to each ABCG2 function. 'Overproduction' hyperuricemia consists of overproduction type and combined type. Full size image Figure 2a shows the association between ABCG2 function and UUE. Contrary to the general understanding that ABCG2 dysfunction leads to decreased renal urate excretion, UUE is significantly increased by ABCG2 dysfunction ( P =3.60×10 −10 ). Whereas the mean UUE level of patients with full ABCG2 function was 24.0 mg h −1 /1.73 m 2 , that of patients with severe dysfunction (≤1/4 function) was 34.3 mg h −1 /1.73 m 2 , showing an increase of 42.9%. The frequency of 'overproduction' hyperuricemia (UUE>25 mg h −1 /1.73 m 2 ), which consists of overproduction type and combined type ( Fig. 1 ), is also increased by ABCG2 dysfunction; the ratio of 'overproduction' hyperuricemia was 38.2% in patients with full function, and reached 89.7% in those with severe dysfunction ( Fig. 2b ). Severe ABCG2 dysfunction especially raised the risk of 'overproduction' hyperuricemia, conferring a risk ratio (RR) of 2.35 (95% CI 1.86–2.97; P =3.32×10 −7 ) ( Table 1 ). In addition, moderate and mild dysfunction also significantly increased the risk of 'overproduction' hyperuricemia, conferring an RR of 1.66 (95% CI 1.32–2.10; P =8.58×10 −6 ) and 1.36 (95% CI 1.09–1.71; P =4.55×10 −3 ), respectively. Risk of overproduction hyperuricemia was still significant after adjustment ( Table 1 ). These results clearly demonstrate that ABCG2 dysfunction increases UUE, thereby leading to increased frequency of 'overproduction' hyperuricemia. This seems paradoxical in light of the current concept of hyperuricemia, but it would be understandable if extra-renal excretion via ABCG2 has a physiologically significant role in urate regulation. Figure 2: Increase of UUE and the frequency of overproduction hyperuricemia by ABCG2 dysfunction. ( a ) UUE according to each ABCG2 function ( n =644). Patients with hyperuricemia were divided into four groups by their estimated ABCG2 functions, that is, full function, 3/4 function, 1/2 function and ≤1/4 function. UUE showed an inverse association with ABCG2 functions ( P =3.60×10 −10 by simple linear regression analysis). All bars show mean±s.e.m. ( b ) Frequency of 'overproduction' hyperuricemia according to each ABCG2 function. 'Overproduction' hyperuricemia consists of overproduction type and combined type. Full size image Table 1 Relationship between overproduction hyperuricemia and ABCG2 dysfunction. Full size table Abcg2 dysfunction and urate excretion in mice Next, we investigated how ABCG2 dysfunction affected the urate excretion pathways and re-evaluated the current concept of hyperuricemia based on ABCG2 dysfunction. The evaluation of gut urate excretion in humans is intrinsically difficult because urate excreted into the intestinal lumen is rapidly metabolized by bacterial flora. To solve this problem, we introduced an animal model in which urate excretion through the gut is easily achievable by invasive sampling. Also, Abcg2 -knockout mice were treated with oxonate, a uricase inhibitor, so that the urate metabolism of this model mimicked that of humans that lacks the urate degrading enzyme, uricase [22] . First, mouse Abcg2 is revealed to mediate urate transport ( Fig. 3a ) using the membrane vesicle system prepared from HEK293 cells that express mouse Abcg2. The export process by mouse Abcg2 was ATP-dependent and not saturable under the physiological concentration of urate ( Fig. 3a ), indicating high-capacity urate transport activity by Abcg2. Another functional analysis demonstrated that oxonate has no hazardous effect on the Abcg2-mediated urate transport ( Fig. 3b ). We then tried to characterize the excretion of urate into urine, bile and intestinal lumen using the in vivo mouse model. As shown in Fig. 3c , SUA of Abcg2 -knockout mice was significantly higher than that of control mice ( P =8.8×10 −6 ), which is consistent with the increase of SUA in humans with ABCG2 dysfunction [21] . Under this condition, the urinary urate/creatinine ratio was significantly increased in Abcg2 -knockout mice ( P =4.1×10 −4 ) ( Fig. 3d ), which also corroborates the observation in humans ( Fig. 2a ). On the other hand, the urate excretion from the intestine was significantly lower in Abcg2 -knockout mice ( Fig. 3e ), which is supported by the similar results of the transintestinal urate transport experiment ( Fig. 3f ; Supplementary Fig. S2 ). Calculated velocity of the intestinal urate excretion in Abcg2 -knockout mice was less than a half of that in control mice ( P =3.6×10 −4 ) ( Fig. 3g ), whereas biliary urate excretion showed no significant difference regardless of Abcg2 genotype ( Fig. 3g ). From these results, we estimated the relative contribution of each pathway to the total urate excretion; in wild-type mice, the UUE pathway contributes approximately two-thirds, and the intestinal excretion pathway contributes one-third of the total urate excretion, whereas the urate excretion into bile is 2.2% of the total urate excretion ( Fig. 3h ). The ratio of each urate excretion pathway is consistent with the previous literature about the estimation of urate excretion pathways in humans [4] , [5] . As a result of decreased intestinal excretion, the urate excretion in Abcg2 -knockout mice was much more dependent on the urinary excretion pathway ( Fig. 3h ). Furthermore, the small contribution of biliary urate excretion in mice ( Fig. 3h ) is also consistent with a report of human urate excretion, which shows that biliary urate excretion consists of less than 5 percent of the total urate excretion [23] . Taken together, ABCG2 is suggested to have an important role in extra-renal urate excretion, especially in intestinal urate excretion. Accordingly, increased SUA in patients with ABCG2 dysfunction can be explained by the decreased excretion of urate from the intestine. 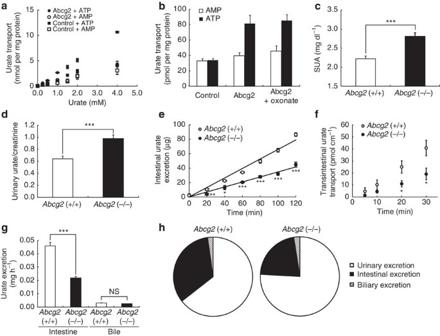Figure 3: Urate excretion via Abcg2 in a mouse model. (a) Concentration-dependent urate transport via Abcg2 (n=3). (b) Effect of oxonate on Abcg2-mediated urate transport (n=3). (c–e,g,h)In vivostudy usingAbcg2-knockout and wild-type mice. (c) Serum uric acid (SUA) levels (n=19–20). ***P=8.8×10−6. (d) Urinary excretion of urate (n=10–11). ***P=4.1×10−4(e) Time course of intestinal urate excretion (n=4). ***P<0.001; **P=0.0066; *P=0.021. (f) Transintestinal urate transport (n=3–4). *P=0.037 and 0.034 for 20 min and 30 min, respectively. (g) Urate excretion in intestine and bile (n=3–4). ***P=3.6×10−4. All bars show means±s.e.m.Pvalues were obtained by Student'st-test. NS, not significant. (h) Relative contribution of urinary, intestinal and biliary urate excretion pathways. Figure 3: Urate excretion via Abcg2 in a mouse model. ( a ) Concentration-dependent urate transport via Abcg2 ( n =3). ( b ) Effect of oxonate on Abcg2-mediated urate transport ( n =3). ( c – e , g , h ) In vivo study using Abcg2 -knockout and wild-type mice. ( c ) Serum uric acid (SUA) levels ( n =19–20). *** P =8.8×10 −6 . ( d ) Urinary excretion of urate ( n =10–11). *** P =4.1×10 −4 ( e ) Time course of intestinal urate excretion ( n =4). *** P <0.001; ** P =0.0066; * P =0.021. ( f ) Transintestinal urate transport ( n =3–4). * P =0.037 and 0.034 for 20 min and 30 min, respectively. ( g ) Urate excretion in intestine and bile ( n =3–4). *** P =3.6×10 −4 . All bars show means±s.e.m. P values were obtained by Student's t -test. NS, not significant. ( h ) Relative contribution of urinary, intestinal and biliary urate excretion pathways. Full size image We found that the decrease in urate exporter ABCG2 function in hyperuricemic patients is associated with the increase of UUE and frequency of overproduction hyperuricemia, which consists of the overproduction type and the combined type. Also, any ABCG2 dysfunction caused by common dysfunctional variants significantly raised the risk of overproduction hyperuricemia. Abcg2 -knockout mice treated with oxonate showed increased renal urate excretion as well as SUA and decreased intestinal urate excretion, compared with those of wild-type mice. These findings indicate that the decrease in extra-renal urate excretion via dysfunctional ABCG2 is a common mechanism of hyperuricemia, which has been currently mistaken for urate 'overproduction' due to increased UUE. Three main transporters have been confirmed to regulate SUA in humans; a secretion transporter ABCG2 and two urate reabsorption transporters, URAT1 (ref. 10 ) and GLUT9 (refs 14 , 15 ). In addition, urate transporters including ABCG2 and URAT1 are regulated by an adaptor protein, the PDZ domain containing-protein, PDZK1 (refs 24 , 25 ). Among these urate-related genes, dysfunctional variants of ABCG2 are demonstrated as a major cause of gout and hyperuricemia [20] , [21] . ABCG2 is expressed on the apical membrane of several tissues including kidney [26] , liver and intestine [27] . As ABCG2 is supposed to mediate renal urate excretion [20] , the dysfunction of this molecule is expected to decrease UUE. The results in this study, however, show an opposite conclusion that the dysfunction of ABCG2 results in an increase of UUE. This contradiction can be explained by two facts: kidney is not the only organ in which ABCG2 is expressed [27] , [28] , and one-third of urate excretion in humans depends on the extra-renal pathway such as gut excretion [4] , [5] , [8] . Also, together with little intestinal expression of URAT1 (ref. 10 ), our data from an animal model indicate that the decreased expression of Urat1 in the kidney could partially account for the increased urate in urine in Abcg2 -knockout mice ( Fig. 3d, Supplementary Fig. S3 ). Therefore, it is reasonable that common dysfunction of ABCG2 can cause a decrease of urate excretion via the extra-renal pathway rather than the renal pathway. The current classification of hyperuricemia is based on the understanding of its mechanism by which hyperuricemia results from either overproduction of urate due to a metabolism disorder, underexcretion by abnormal renal urate transport activity, or the combination of the two. So far 'renal urate underexcretion' has been widely considered to be a main cause of hyperuricemia, and 'urate overproduction' is recognized as another common cause. A part of hyperuricemia is definitely attributable to lifestyle factors such as consumption of an excessive amount of alcohol as well as high-calorie diet intake. However, even taking such factors into account, most causes of 'overproduction' hyperuricemia still cannot be explained. Many attempts have been made to elucidate the pathogenesis of 'overproduction' hyperuricemia. Nevertheless, no study has succeeded in identifying the exact mechanism of urate overproduction except some urate metabolism disorders [29] including Lesch–Nyhan syndrome (hypoxanthine-guanine phosphoribosyl transferase deficiency), accelerated purine nucleotide degradation and accelerated ATP breakdown. Our findings indicate that a major cause of 'overproduction' hyperuricemia is not true overproduction of urate but rather 'extra-renal urate underexcretion' by common ABCG2 dysfunction. We also suggest that re-classification of hyperuricemia is necessary because 'overproduction' hyperuricemia in the current classification is only defined by the result of UUE value and does not represent a correct pathophysiological condition. Therefore, our data lend support to the idea that 'overproduction type' in the current classification of hyperuricemia should be renamed 'renal overload type,' which includes subtypes of 'extra-renal underexcretion' and genuine 'overproduction' ( Fig. 4 ). 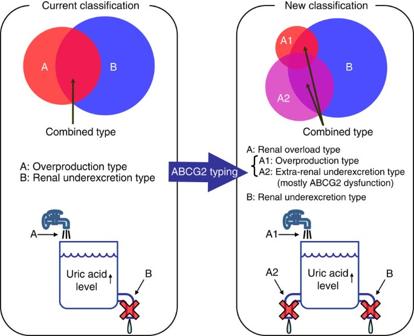Figure 4: Pathophysiological model and proposed new classification of hyperuricemia. Hyperuricemia is currently classified into urate 'overproduction type' (A), 'renal underexcretion type' (B), and combined type. Taking extra-renal urate excretion into account, we propose a testable model by which 'overproduction type' be renamed 'renal overload type' (A), consisting of two subtypes, genuine 'overproduction' (A1) and 'extra-renal underexcretion' (A2). Figure 4: Pathophysiological model and proposed new classification of hyperuricemia. Hyperuricemia is currently classified into urate 'overproduction type' (A), 'renal underexcretion type' (B), and combined type. Taking extra-renal urate excretion into account, we propose a testable model by which 'overproduction type' be renamed 'renal overload type' (A), consisting of two subtypes, genuine 'overproduction' (A1) and 'extra-renal underexcretion' (A2). Full size image In this study, we suggest a common mechanism of hyperuricemia by decreased extra-renal excretion due to ABCG2 dysfunction. Therefore, ABCG2 could be a promising target for urate-lowering medications without adverse effects such as urolithiasis. Our findings and proposal would serve to correct the long-misunderstood pathophysiology of hyperuricemia. This new concept will help pinpoint the causes of hyperuricemia more accurately and provide a more effective therapeutic strategy for hyperuricemia and gout, leading to a good model of personalized medicine for common diseases. Study participants This study was approved by the institutional ethical committees, and all procedures involved in this study were performed in accordance with the Declaration of Helsinki. Hyperuricemia patients were diagnosed when their SUAs were higher than 7.0 mg dl −1 , and gout cases were also clinically diagnosed as primary gout according to the criteria established by the American College of Rheumatology [30] . All hyperuricemic subjects and primary gouty patients were eligible, when written consent was obtained at the gout clinics of either Jikei University Hospital (Tokyo, Japan) or Midorigaoka Hospital (Osaka, Japan). The following patients were excluded; patients without information on clinical parameters shown in Supplementary Table S1 , or those with inherited metabolism disorders including Lesch–Nyhan syndrome. Finally, 644 male outpatients, including 575 gout cases, were registered as valid participants. Clinical parameters for urate handling Clinical parameters including SUA, amount of UUE and fractional excretion of urate clearance (urate clearance/creatinine clearance ratio, FE UA ) were measured for each patient after diet education, concerning low-purine and calorie-controlled diet, as well as less fructose and alcohol intake [31] , [32] . Clinical parameters before taking medications for hyperuricemia were used in this study. Both UUE and FE UA were calculated after a few-hour urine collection. UUE was normalized for a body surface area of 1.73 m 2 . In this study, patients were classified as overproduction hyperuricemia when their UUE was over 25.0 mg h −1 /1.73 m 2 (600 mg day −1 /1.73 m 2 ) [7] , [8] , [33] . Those who had FE UA under 5.5% were classified as underexcretion hyperuricemia [34] on the basis of the normal FE UA range (5.5–11.1%) [35] . Combined type was classified when their UUE and FE UA met the criteria of both overproduction and underexcretion hyperuricemia ( Fig. 1 ). Patients who met the single criterion of overproduction hyperuricemia, excluding combined type, were defined as overproduction type. Genetic analysis Genomic DNA was extracted from whole peripheral blood cells [36] . Genotyping was performed by high-resolution melting analysis with a LightCycler 480 (Roche Diagnostics) [21] , or by an allelic discrimination assay (Custom Taqman MGB, Applied Biosystems) with a 7700 detector (Applied Biosystems) [37] . To confirm their genotypes, more than 100 samples were subjected to direct sequencing with primers shown in Supplementary Table S5 . DNA sequencing analysis was performed with a 3130×l Genetic Analyzer (Applied Biosystems) [21] . The export function of ABCG2 was then estimated from the combinations of ABCG2 variants, rs72552713 (Q126X) and rs2231142 (Q141K), and divided into four functional groups [21] ; that is, full function, 3/4 function (mild dysfunction), 1/2 function (moderate dysfunction) and ≤1/4 function (severe dysfunction). Experimental assessment for urate excretion pathways Mouse Abcg2 complementary DNA (GenBank accession number NM_011920 ) was inserted into the Not I site of pcDNA3.1(+) vector plasmid (Invitrogen), with a myc-tag sequence attached at the 5′-end. The wild-type human ABCG2 cDNA (GenBank accession number NM_004827 ) or mutated (Q126X and Q141K) ABCG2 cDNA was inserted into the Nhe I and Apa I sites of pcDNA3.1(+) vector plasmid, with a myc-tag sequence attached at the 5′-end [21] . To prepare membrane vesicles, HEK293 cells were transiently transfected with the expression vector for Abcg2/ABCG2 or empty vector (control) by FuGENE6 (Roche Diagnostics), according to the manufacturer's instructions. Forty-eight hours later, cells were collected and the membrane vesicles were isolated by a standard method with repeated centrifugation and homogenization [38] . After the expression of Abcg2 protein was confirmed by western blot analysis, the uptake studies of [ 14 C]urate (28 μM, American Radiolabeled Chemicals) were performed by a standard protocol for transport assays with membrane vesicles [39] . All other chemicals used in this study were commercially available and of reagent-grade. Male Abcg2 -knockout mice (FVB.129P2-Abcg2, Taconic) and control FVB mice of 27–33 g were fed 2.0% (w/w) potassium oxonate for more than 1 week, as reported earlier [40] . Concentrations of urate and creatinine in collected serum and urine samples were determined by QuantiChrom Uric Acid Assay Kit (Bioassay systems) and Creatinine Assay Kit (Cayman Chemical Company). To analyze the intestinal urate excretion, mice fasted-overnight were anaesthetized by intraperitoneal injection of urethane and cannulated with polyethylene tubing (Hibiki Size 8) (Kunii Co.) at the upper duodenum and the middle jejunum to make an intestinal loop at the upper half of the intestine. After the intestinal contents were removed by the slow infusion of saline and air, the efflux buffer (saline containing 0.3 mM potassium oxonate) was introduced into the intestinal loop, and both ends of the loop were closed with syringes. After the indicated periods, the efflux buffer in the loop was collected by syringes and urate concentrations were quantified. Intestinal urate excretion was calculated from the following equation: To investigate the biliary urate excretion, mice were anaesthetized by intraperitoneal injection of urethane, the cystic duct was ligated and a common bile duct fistula was created using a Teflon catheter (UT-03) (Unique Medical). Urate in the hepatic bile specimens collected for 3 h was examined. Relative contribution of urinary, intestinal and biliary excretion pathways was estimated by the comparison of the calculated velocity of each pathway, for which the amount of daily urine is assumed to be 2 millilitres. Protocols were performed according to accepted criteria for humane care of experimental animals and approved by the review board of our institution for animal studies. Western blot analysis For western blot analysis, 5 μg of membrane vesicles diluted with 2×SDS loading buffer was separated on a 10% SDS-polyacrylamide gel electrophoresis plate with a 3.75% stacking gel. Proteins were transferred electrophoretically onto an Immunobilon membrane (Millipore) using a blotter (Bio-Rad Laboratories) at 15 V for 1 h. The membrane was blocked with Tris-buffered saline containing 0.05% Tween 20 (TBS-T) and 3% bovine serum albumin (BSA) for 1 h at room temperature. After washing with TBS-T, the membrane was incubated for 1 h at room temperature in TBS-T containing 0.1% BSA and anti-ABCG2/BCRP antibody (BXP-53, Abcam) (1:500, 0.5 μg ml −1 ) for the detection of ABCG2, or anti-Na+/K+-ATPase α antibody (Santa Cruz Biotechnology) (1:200, 1.0 μg ml −1 ) as a loading control of membrane proteins. For detection, the membrane was allowed to bind to a horseradish peroxidase-labelled secondary antibody (GE Healthcare) diluted 5,000-fold in TBS-T containing 0.1% BSA for 1 h at room temperature. The enzyme activity was assessed using an ECL Prime Western Blotting Detection System (GE Healthcare) with a luminescent image analyzer (Bio-Rad). Transintestinal urate transport experiment To demonstrate the intestinal transport of urate, the upper third of mice intestine specimens was collected and enteral contents were carefully removed. Next, both ends of the specimens were connected with syringes and the luminal sides were filled with 5 ml of Ringer Buffer (93.4 mM NaCl, 6.2 mM KCl, 2.0 mM KH 2 PO 4 , 1.2 mM MgSO 4 -7H 2 O, 2.5 mM CaCl 2 -2H 2 O, pH 7.4, 37 °C). Then, the specimens were incubated with [ 14 C]urate (0.4 μM)-containing Ringer Buffer (pH 7.4, 37 °C), pre-bubbled with mixed gas (95% O 2 and 5% CO 2 ) for 30 min. After incubation with indicated periods, 200 μl of luminal buffer was sampled followed by the addition of the same aliquot of the buffer. Syringes were slowly pumped every 2.5 min to thoroughly mix the luminal buffer ( Supplementary Fig. S2 ). Quantitative real-time PCR To determine messenger RNA levels of genes involved in urate transport, mice kidney specimens were homogenized in RNA iso plus (Takara) and extracted RNA was reverse-transcribed with ReverTra Ace (Toyobo). Quantitative real-time PCR was performed using 2× SYBR GREEN (Stratagene) and Chromo4 (BIO-RAD) at 95 °C 10 min followed by 40 cycles at 95 °C for 15 s, 50 °C for 30 s, and 72 °C for 40 s. We used primers for Abcg2 (sense and antisense primers were 5′-aagcatagggatggagctga-3′ and 5′-ctgtgcttgagtccaaacca-3′, respectively), Urat1 (sense and antisense primers were 5′-atcatctccatgctgtgctg-3′ and 5′-aagtccacaatcccgatgag-3′, respectively), Glut9 (sense and antisense primers were 5′-cggcctggctctcaaacttcgccg-3′ and 5′-ggcgaagacgaggaagcagt-3′, respectively), Pdzk1 (sense and antisense primers were 5′-atataatgcctcagggcgtg-3′ and 5′-atggctggcgttctctacat-3′, respectively) and β-actin (sense and antisense primers were 5′-ccggaaggaaaactgacagc-3′ and 5′-gtggtggtgaagctgtagcc-3′, respectively). Statistical analysis Haplotype estimation was performed with the EM algorithm [41] . To investigate the association of ABCG2 functions and UUE, simple linear regression analysis was performed with UUE as a dependent variable and estimated function of ABCG2 as an independent variable. To evaluate the relationship between ABCG2 function and overproduction hyperuricemia, the risk ratio (RR) and its 95% CI were calculated by dividing the proportion of overproduction hyperuricemia in each function category by that in full function category. Poisson regression analysis was performed to obtain adjusted RR of ABCG2 dysfunction for overproduction hyperuricemia with possible confounding factors, such as body mass index, alcohol intake, single nucleotide polymorphisms of urate-related genes, rs11722228 ( GLUT9 / SLC2A9 ) [18] , rs506338 ( URAT1 / SLC22A12 ) [18] , and rs12129861( PDZK1 ) [17] . For all calculations in the statistical analysis, software R (version 2.8.1) ( http://www.r-project.org/ ) and SPSS (version 16.0J for Windows) (SPSS) were used. How to cite this article: Ichida, K. et al . Decreased extra-renal urate excretion is a common cause of hyperuricemia. Nat. Commun. 3:764 doi: 10.1038/ncomms1756 (2012).